Disorder-induced topological change of the superconducting gap structure in iron pnictides In superconductors with unconventional pairing mechanisms, the energy gap in the excitation spectrum often has nodes, which allow quasiparticle excitations at low energies. In many cases, such as in d -wave cuprate superconductors, the position and topology of nodes are imposed by the symmetry, and thus the presence of gapless excitations is protected against disorder. Here we report on the observation of distinct changes in the gap structure of iron–pnictide superconductors with increasing impurity scattering. By the successive introduction of nonmagnetic point defects into BaFe 2 (As 1− x P x ) 2 crystals via electron irradiation, we find from the low-temperature penetration depth measurements that the nodal state changes to a nodeless state with fully gapped excitations. Moreover, under further irradiation the gapped state evolves into another gapless state, providing bulk evidence of unconventional sign-changing s -wave superconductivity. This demonstrates that the topology of the superconducting gap can be controlled by disorder, which is a strikingly unique feature of iron pnictides. When repulsive electron–electron interactions are strong, a sign change in the superconducting order parameter (or the gap function) often leads to some energy gain for electron pairing [1] , [2] . The positions of the gap nodes in momentum k space, at which the order parameter changes sign, are determined by the superconducting pairing interactions. In the high transition temperature ( T c ) cuprates, it has been established that the lines of nodes are located along k x =± k y , as expected from the symmetry of the order parameter [3] . In iron pnictides, on the other hand, the multiband Fermi surface structure leads to several candidates for the superconducting symmetry, including sign-changing s ± with and without nodes, sign-preserving s ++ , d -wave and time-reversal symmetry breaking s + id (refs 2 , 4 , 5 , 6 , 7 , 8 , 9 , 10 ). Different symmetries and details of higher order momentum dependence of the gap yield topologically different nodal structures such as vertical or horizontal lines of nodes, nodal loops or no nodes. The effect of nonmagnetic impurities on unconventional superconductivity has been one of the central issues in condensed matter physics [11] , [12] . For the conventional Bardeen-Cooper-Schrieffer (BCS) superconductors, it has been established that the effect is essentially null: the transition temperature is robust against nonmagnetic impurity scattering (the so-called Anderson theorem) and so is the superconducting gap. For the unconventional superconductors, one of the important aspects of the impurity effects is to mix gaps on different parts of the Fermi surface and thereby smear out the momentum dependence [13] . In the case of superconducting gap with symmetry protected nodes such as d -wave, this averaging mechanism leads to the suppression of the gap amplitude, which enhances the low-lying quasiparticle excitations near the nodal positions. In addition to this, the sign change in the order parameter gives rise to impurity-induced Andreev bound states, which lead to additional quasiparticle excitations [14] . Such pair-breaking effects of nonmagnetic impurities have been observed, for example, in Zn-doped YBa 2 Cu 3 O 7 in the bulk measurements of magnetic penetration depth, where the T -linear temperature dependence in the clean-limit d -wave superconductivity gradually changes to a T 2 dependence at low temperatures with increasing Zn concentrations [15] . In sharp contrast, when the nodal positions are not symmetry protected, as in the nodal s -wave case, the averaging mechanism of impurity scattering can displace the nodes, and at a certain critical impurity concentration the nodes may be lifted if intraband scattering dominates [13] , eliminating the low-energy quasiparticle excitations. In the fully gapped state after the node lifting, we have two cases in the multiband superconductors. If the signs of the order parameter on different bands are opposite, residual interband scattering can give rise to midgap Andreev bound states localized at nonmagnetic impurities that can contribute to the low-energy excitations, provided that the concentration of impurities is enough to create such states. If there is no sign change, the gap and T c will be disorder independent after a sufficient amount of impurity scattering: no Andreev states will be created, and thus no significant further change of the low-energy excitations is expected. Indeed, such a difference between nodal sign-changing s ± and sign-preserving s ++ cases has been theoretically suggested by the recent calculations for multiband superconductivity, considering the band structure of iron pnictides [16] . Therefore, the impurity effects on the gap nodes and low-energy excitations can be used as a powerful probe for the pairing symmetry of superconductors. Here we demonstrate, by using electron irradiation to control disorder, that the low-energy excitations show two-step changes with increasing impurity scattering in an iron–pnictide superconductor. This successive evolution of the superconducting gap structure, which has not been observed previously, provides compelling bulk evidence for the sign-changing s ± symmetry of the superconducting order parameter. Disorder effects on superconducting transition In this study, we focus on the isovalently substituted system BaFe 2 (As 1− x P x ) 2 close to the optimum composition with T c ~30 K (ref. 17 ). This system is particularly suitable for the study of the impurity effect on gap structure, because several experiments have indicated that the pristine crystals are very clean and exhibit nodes in the superconducting gap [18] . To detect changes in the low-energy quasiparticle excitations, we measure the magnetic penetration depth λ at low temperatures, a fundamental property of superconductors whose T -dependence is directly related to the excited quasiparticles. Tunnel diode oscillators (TDOs) [19] , [20] in 3 He and dilution refrigerators operating at 13 MHz are used to measure the temperature dependence of λ down to 0.4 K and 80 mK, respectively [21] , [22] . The frequency shift of the TDO is also used to determine the bulk superconducting transition of each crystal. To introduce the impurity scattering in a controllable way, we employ electron irradiation with incident energy of 2.5 MeV, for which the energy transfer from the impinging electron to the lattice is above the threshold energy for the formation of vacancy-interstitial (Frenkel) pairs that act as point defects. The long attenuation length and the small recoil energy due to the small mass of electrons is important to create uniformly distributed point defects over the entire crystal with the width of ~30 μm ( Fig. 1a–d ). If the recoil energy is too large, one may expect creation of complex defects such as clusters and cascades of point defects and, in the extreme case, columnar tracks, which has been realized by heavy-ion irradiation [23] ( Fig. 1b,c ). Another advantage of electron irradiation is that, unlike chemical substitutions, the defects can be introduced without changing lattice constants, which is quite important as the gap structure may be sensitive to the lattice parameters in iron-based superconductors [2] . 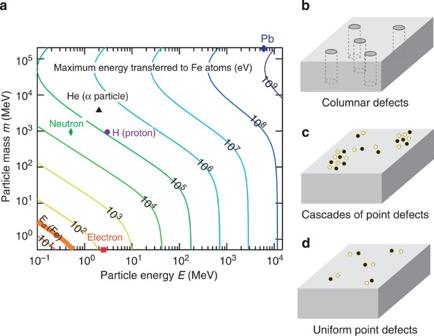Figure 1: Particle irradiation and created defects. (a) Contour plot of maximum energy transferred to Fe atoms (recoil energy) for irradiated particles with the rest massmand incident energyE. Typical threshold energyEdfor the displacement of Fe atoms from the lattice is marked by thick orange line. Typical energies for electron (red square), neutron (green diamond), proton (purple circle), α particle (black triangle) and heavy-ion Pb (blue diamond) irradiation are indicated. Owing to its small mass, the recoil energy of the electron irradiation used in this study is orders of magnitude smaller than those of other particle cases. (b–d) Schematic illustrations for different types of defects created by particle irradiation. Columnar defects can be created by heavy-ion irradiation (b). Particle irradiation with relatively large recoil energies tends to have cascades of point defects due to successive collision of atoms (c). Electron irradiation with a small recoil energy is the most reliable way to obtain uniform point defects (d). Figure 1: Particle irradiation and created defects. ( a ) Contour plot of maximum energy transferred to Fe atoms (recoil energy) for irradiated particles with the rest mass m and incident energy E . Typical threshold energy E d for the displacement of Fe atoms from the lattice is marked by thick orange line. Typical energies for electron (red square), neutron (green diamond), proton (purple circle), α particle (black triangle) and heavy-ion Pb (blue diamond) irradiation are indicated. Owing to its small mass, the recoil energy of the electron irradiation used in this study is orders of magnitude smaller than those of other particle cases. ( b – d ) Schematic illustrations for different types of defects created by particle irradiation. Columnar defects can be created by heavy-ion irradiation ( b ). Particle irradiation with relatively large recoil energies tends to have cascades of point defects due to successive collision of atoms ( c ). Electron irradiation with a small recoil energy is the most reliable way to obtain uniform point defects ( d ). Full size image By successive electron irradiation into clean single crystals of BaFe 2 (As 1− x P x ) 2 , x =0.33–0.36, with initial transition temperatures T c0 of 28, 29 and 30 K, we observe a systematic downward shift of T c with increasing defect dose ( Fig. 2a–d ). The transition width in the TDO frequency change ( Fig. 2a,b ) remains almost unchanged after irradiation, which implies a good homogeneity of the point defects introduced. The temperature dependence of in-plane resistivity ρ ( T ) measured by the van der Pauw configuration ( Fig. 2c ) shows parallel shifts of ρ ( T ) after each irradiation in a single crystal. The parallel shifts imply that point defects increase impurity (elastic) scattering with little change of carrier concentrations and inelastic scattering, which is closely related to the electron correlations. 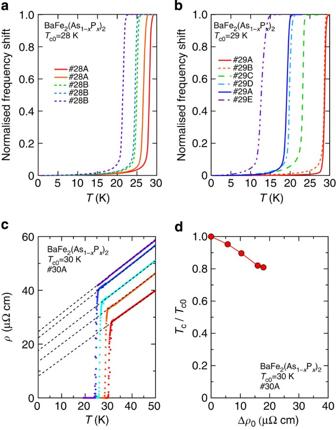Figure 2: Effect of electron irradiation on the superconducting transition in BaFe2(As1−xPx)2single crystals. (a) Temperature dependence of the TDO frequency shift normalized by the total shift during the superconducting transitions for crystals (#28A and #28B) from a batch ofTc0=28 K with irradiated doses of 0, 1.0, 2.0, 4.0 and 6.0 C cm−2with decreasingTc. (b) Similar plot for crystals (#29A, #29B, #29C, #29D and #29E) from a batch ofTc0=29 K with irradiated doses of 0, 1.5, 2.7, 4.7, 4.9 and 8.3 C cm−2with decreasingTc. (c) Temperature dependence of resistivity for a crystal (#30A) withTc0=30 K with irradiated doses of 0, 1.1, 2.3, 3.8 and 4.5 C cm−2with decreasingTc. Dotted lines are linear extrapolations to zero temperature to estimate changes in residual resistivity Δρ0. (d) Transition temperatureTcnormalized by the pristine valueTc0=30 K as a function of Δρ0, determined by the resistivity measurements in crystal #30A. Figure 2: Effect of electron irradiation on the superconducting transition in BaFe 2 (As 1− x P x ) 2 single crystals. ( a ) Temperature dependence of the TDO frequency shift normalized by the total shift during the superconducting transitions for crystals (#28A and #28B) from a batch of T c0 =28 K with irradiated doses of 0, 1.0, 2.0, 4.0 and 6.0 C cm −2 with decreasing T c . ( b ) Similar plot for crystals (#29A, #29B, #29C, #29D and #29E) from a batch of T c0 =29 K with irradiated doses of 0, 1.5, 2.7, 4.7, 4.9 and 8.3 C cm −2 with decreasing T c . ( c ) Temperature dependence of resistivity for a crystal (#30A) with T c0 =30 K with irradiated doses of 0, 1.1, 2.3, 3.8 and 4.5 C cm −2 with decreasing T c . Dotted lines are linear extrapolations to zero temperature to estimate changes in residual resistivity Δ ρ 0 . ( d ) Transition temperature T c normalized by the pristine value T c0 =30 K as a function of Δ ρ 0 , determined by the resistivity measurements in crystal #30A. Full size image We estimate the change in the residual resistivity Δ ρ 0 by extrapolating the normal state data linearly to zero temperature. The T c reduction rate with respect to Δ ρ 0 is about −0.3 K μΩ −1 cm −1 ( Fig. 2d ), which is comparable to the similar electron irradiation measurements in Ru-substituted BaFe 2 As 2 (ref. 24 ). Previous studies of the T c reduction rate in iron–pnictide superconductors by chemical substitutions [25] , [26] , [27] and by particle irradiation [24] , [28] , [29] , [30] focus on the comparisons with theoretical calculations for s ± and s ++ -wave superconductivity [16] , [31] , but they report various values of the suppression rate. Here we instead focus on changes of low-energy excitations induced by disorder from penetration depth measurements. Previously, the disorder effect of the penetration depth has been reported in Ba(Fe, T ) 2 As 2 ( T =Co, Ni) (refs 32 , 33 ) and (Ba,K)Fe 2 As 2 (refs 34 , 35 ) for the cases of natural disorder [34] and columnar defects introduced by heavy-ion irradiation [32] , [33] , [35] , but the effect of controlled point defects, which can be compared closely to the theoretical calculations, has been lacking. Disorder effects on penetration depth In pristine crystals of BaFe 2 (As 1− x P x ) 2 , the penetration depth shows a strong temperature dependence at low temperatures ( Fig. 3a,b ), as reported previously [21] , [22] . The temperature dependence of the change in the penetration depth Δ λ ( T )= λ ( T )− λ (0) can be fitted to a power law T n with the exponent n <1.5, indicating that this system has line nodes in the energy gap. After irradiation, we first find that Δ λ ( T ) at the lowest temperatures becomes more gentle, or the exponent n increases, and in the T c0 =28 K crystal we have almost T 2 dependence ( Fig. 3a ). Further increase of the defect density results in a flat temperature dependence below T / T c ~0.06–0.1, indicating that the system is changed to a fully gapped state ( Fig. 3c,d ). A fitting to the exponential dependence gives the gap size 2Δ ≳ k B T c , which is a substantial portion of the BCS value. Such flat temperature dependence of Δ λ has been reproduced in three crystals measured in this study, one of which has been measured down to 80 mK ( Fig. 3e ). The data represent completely temperature-independent behaviour below T / T c ~0.05 within a precision of ~1 Å ( Fig. 3e , inset). 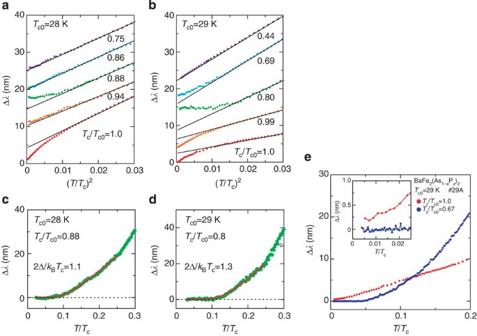Figure 3: Effect of electron irradiation on the low-temperature penetration depth in BaFe2(As1−xPx)2single crystals. (a,b) Change in the magnetic penetration depth Δλplotted against (T/Tc)2for the sameTc0=28 K samples asFig. 2a(a) and for theTc0=29 K samples asFig. 2b(b). The same colours are used asFig. 2a,bfor the corresponding irradiated doses. Each curve is shifted vertically for clarity. Lines are theT2dependence fits at high temperatures. (c,d) Temperature dependence of Δλfor sample #28B with 2.0 C cm−2(c) and for sample #29C with 2.7 C cm−2(d). Red lines are the fits to the exponential dependence expected in fully gapped superconductors. (e) Temperature dependence of Δλfor sample #29A before (red) and after irradiation (blue) of 4.9 C cm−2dose. Inset is an expanded view at the lowest temperatures. Figure 3: Effect of electron irradiation on the low-temperature penetration depth in BaFe 2 (As 1− x P x ) 2 single crystals. ( a , b ) Change in the magnetic penetration depth Δ λ plotted against ( T / T c ) 2 for the same T c0 =28 K samples as Fig. 2a ( a ) and for the T c0 =29 K samples as Fig. 2b ( b ). The same colours are used as Fig. 2a,b for the corresponding irradiated doses. Each curve is shifted vertically for clarity. Lines are the T 2 dependence fits at high temperatures. ( c , d ) Temperature dependence of Δ λ for sample #28B with 2.0 C cm −2 ( c ) and for sample #29C with 2.7 C cm −2 ( d ). Red lines are the fits to the exponential dependence expected in fully gapped superconductors. ( e ) Temperature dependence of Δ λ for sample #29A before (red) and after irradiation (blue) of 4.9 C cm −2 dose. Inset is an expanded view at the lowest temperatures. Full size image The fact that we do not observe any Curie upturn at low temperatures is a strong indication that the point defects are essentially nonmagnetic. In the presence of magnetic impurities, the TDO frequency shift has a contribution from the paramagnetic susceptibility term and thus is proportional to Δ λ ( T )+2 λ (0) nμ 0 μ 2 /(3 V cell k B T ) [36] , [37] , where n and μ are the density and the effective moment of the magnetic impurity, μ 0 is the vacuum permeability, and V cell is the unit-cell volume containing four Fe atoms. If we use an estimate of the defect density [38] and the reported value of λ (0)≈0.2 μm [22] , our precision of the measurement on the sample #29A with the irradiated dose of 4.9 C cm −2 ( Fig. 3e ) gives an upper limit on the magnetic moment of ~0.2 μ B per Fe defect. This is much smaller than the spin moment of 4.9 μ B expected in the magnetic state of a free Fe 2+ ion. The exact numbers of local moments of magnetic defects inside the iron–pnictide materials are difficult to estimate, but recent X-ray emission spectroscopy measurements revealed that the instantaneous local moments in various iron pnictides are always about 1 μ B per Fe, and for the BaFe 2 As 2 case ~1.3 μ B per Fe has been found [39] . Thus it is expected that the moment of the order of 1 μ B per defect would appear if the defects act as magnetic impurities, which can be ruled out by our results of the lack of a Curie upturn within the ~0.2 μ B resolution. Further increase of the defect density leads to another change of Δ λ ( T ). The T -dependence at the lowest temperatures gets steeper with increasing defect dose, which is an opposite trend to the initial change at low doses. This second stage of changes clearly indicates that by irradiation we create low-energy excitations again inside the formed gap. At the highest doses we measured, we observe the T 2 dependence, which is a manifestation of the formation of the Andreev bound states expected for the sign-changing order parameter with impurity scattering. The impurity band corresponding to these bound states must overlap the Fermi level to cause this effect. We should also point out that in this second stage we still observe a strong reduction of T c with irradiation ( Fig. 2a,b ). This is clearly different from the expectation of the conventional s -wave case without sign reversal, which further supports the presence of sign change in the order parameter after the node lifting. The observation of the impurity-induced fully gapped state provides one of the strongest pieces of evidence from bulk measurements that the nodes are not symmetry protected in this system. Moreover, the two-stage changes in the low-energy excitations observed here most likely come from the peculiar band-dependent gap functions of multiband iron-pnictide superconductors. Owing to the well-separated hole and electron Fermi surface sheets, fully gapped s ± superconductivity with opposite signs of the order parameter on different bands has been predicted by the theories based on spin fluctuations with the antiferromagnetic vector Q =( π , π ) in the two-Fe zone notation [4] , [5] . The presence of nodes in the pristine samples implies some competing additional mechanisms, such as spin fluctuations with a different Q vector [5] , anisotropic Fermi surface orbital weights [7] , or orbital fluctuations, which prefer the same sign in both bands [8] , [9] . To reproduce the observed two-stage changes, we have made calculations for the low-energy excitations and the low-temperature behaviour of λ ( T ) by using a two-band model [16] ( Fig. 4a–d ). We assume that one band is fully gapped, and the other has accidental nodes whose positions are not symmetry protected. Two possible realizations with s ± and s ++ structure are shown in Fig. 4a . 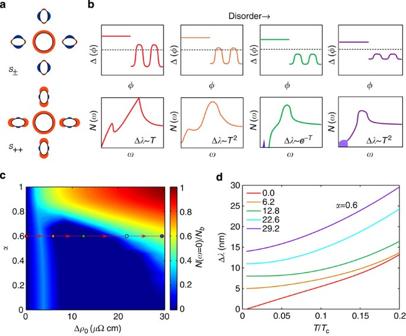Figure 4: Theoretical calculations of impurity effects in iron-based superconductors. (a) Schematic of possibles±ands++states. Large circles and small ellipsoids (black lines) are hole and electron Fermi surfaces, respectively. Red and blue represents the superconducting order parameter with different signs. (b) Schematic ofs±order parameter versus azimuthal angleφ(top row) and density of statesNversus energyω(bottom row) with increasing irradiation dosage (from left to right). Dotted lines (top row) are zero lines. (c) Density of states at Fermi levelN(0) for nodal band plotted as false colour versus inter to intraband scattering ratioαand irradiation-induced residual resistivity Δρ0for the model defined in the study by Wanget al.16(d) Penetration depth change Δλversus reduced temperatureT/Tcfor different values of Δρ0as marked in legend, and inter to intraband scattering ratioα=0.6 (arrows inc). Each curve is shifted vertically for clarity. Figure 4b shows schematically the evolution of the gap function in the s ± case as a function of increasing disorder of dominant intraband and subdominant interband character. The corresponding densities of states are also plotted. Only in the last panels, where the subgap bound state appears, do the s ± and s ++ cases differ qualitatively. Figure 4: Theoretical calculations of impurity effects in iron-based superconductors. ( a ) Schematic of possible s ± and s ++ states. Large circles and small ellipsoids (black lines) are hole and electron Fermi surfaces, respectively. Red and blue represents the superconducting order parameter with different signs. ( b ) Schematic of s ± order parameter versus azimuthal angle φ (top row) and density of states N versus energy ω (bottom row) with increasing irradiation dosage (from left to right). Dotted lines (top row) are zero lines. ( c ) Density of states at Fermi level N (0) for nodal band plotted as false colour versus inter to intraband scattering ratio α and irradiation-induced residual resistivity Δ ρ 0 for the model defined in the study by Wang et al . [16] ( d ) Penetration depth change Δ λ versus reduced temperature T / T c for different values of Δ ρ 0 as marked in legend, and inter to intraband scattering ratio α =0.6 (arrows in c ). Each curve is shifted vertically for clarity. Full size image Figure 4c,d shows concrete theoretical calculations using the model of Wang et al . [16] in support of this scenario. The variation of the density of states at the Fermi level with scattering rate and the ratio α of inter and intraband scattering ( Fig. 4c ), clearly shows the nonmonotonic behaviour of the density of states with scattering rate at a fixed α . The temperature dependence of Δ λ depends directly on the residual density of states at the Fermi level, and therefore changes with increasing scattering as follows: (1) T -linear, (2) T 2 , (3) exponential and (4) T 2 ( Fig. 4d ). It is the overlap of the bound state in the last panel—not present in the s ++ case—with the Fermi level that gives rise to the ‘re-entrant’ final T 2 dependence of the penetration depth. Thus the observed sequential changes of Δ λ ( T ) in this system are fully consistent with a sign-changing s -wave superconducting gap of s ± type. Our results demonstrate that the gap topology and the low-energy excitations can be changed by controlling disorder. Such an impurity effect is unprecedented among superconductors, highlighting a unique aspect of iron-based superconductors. Our study also shows that the impurity effects on gap structure can provide phase information on the superconducting order parameter in bulk measurements, in contrast to other phase sensitive experiments [3] , [40] , most of which require excellent surfaces or interfaces. Single crystals Single crystals of BaFe 2 (As 1− x P x ) 2 were grown by the self-flux method [17] and characterized by several techniques as reported previously [18] . The observation of the quantum oscillations in this series of crystals and the sharp superconducting transition indicate the very high quality of our pristine crystals. We used several crystals from three batches, which exhibit slightly different T c0 values of 28, 29 and 30 K. Typical dimensions of the crystals are (200–300) × (200–300) × ~30 μm 3 . Experimental techniques Electron irradiation experiments were performed on SIRIUS platform operated by Laboratoire des Solides Irradies (LSI) at Ecole Polytechnique, composed by the Pelltron type NEC accelerator and a closed cycle cryocooler, maintaining the sample immersed in liquid hydrogen at 20–22 K during irradiation. The low-temperature environment is important to prevent defect migration and agglomeration. Partial annealing of the introduced defects occurs upon warming to room temperature and during the sample transfer [24] . The resistivity measurements were performed at LSI, Ecole Polytechnique by the van der Pauw method with four contacts on corners of crystals to minimize the possible effect of the unirradiated area due to contacts. The penetration depth measurements by using 13 MHz TDOs [21] , [22] were performed at Kyoto University before and after irradiation. How to cite this article: Mizukami, Y. et al . Disorder-induced topological change of the superconducting gap structure in iron pnictides. Nat. Commun. 5:5657 doi: 10.1038/ncomms6657 (2014).